Impact of the Mertz Glacier Tongue calving on dense water formation and export Antarctic Bottom Water (AABW) is a critical component of the global climate system, occupying the abyssal layer of the World Ocean and driving the lower limb of the global meridional overturning circulation. Around East Antarctica, the dense shelf water (DSW) precursor to AABW is predominantly formed by enhanced sea ice formation in coastal polynyas. The dominant source region of AABW supply to the Australian–Antarctic Basin is the Adélie and George V Land coast, in particular, polynyas formed in the western lee of the Mertz Glacier Tongue (MGT) and the grounded iceberg B9b over the Adélie and the Mertz Depressions, respectively. The calving of the MGT, which occurred on 12–13 February 2010, dramatically changed the environment for producing DSW. Here, we assess its impact using a state-of-the-art ice-ocean model. The model shows that oceanic circulation and sea ice production in the region changes immediately after the calving event, and that the DSW export is reduced by up to 23%. The oceanic global thermohaline circulation transports a large amount of heat from low to high latitudes and between the two hemispheres, having an important role in controlling the long-term stability and variability of the climate [1] , [2] . It is driven by the sinking of dense water in both polar regions [3] . Antarctic Bottom Water (AABW), which forms from dense shelf water (DSW) overflows in several regions around the Antarctic margin, occupies the abyssal layer of the World Ocean [4] . Assessing the sensitivity of AABW production and its contribution to the global thermohaline circulation is critical, because of the predicted impacts of a reduction/shutdown on the global climate system [5] , [6] . It is recently reported that the bottom layer of the North Pacific Ocean has been warming, possibly because of a slowdown of the Pacific meridional overturning circulation [7] , [8] , [9] , [10] , [11] . There is observational evidence that the overflows of DSWs formed off the Adélie and George V Land coast of East Antarctica predominantly supplies the bottom layer water in the Australian–Antarctic Basin [12] , [13] . Numerical simulation further indicates that this water accounts for a significant part of the bottom layer water in the North Pacific Ocean [14] , [15] . In the Adélie and George V Land region ( Fig. 1 ) the combination of the wind regime and the blocking features of the floating Mertz Glacier Tongue (MGT) and nearby grounded icebergs created a polynya system [16] , [17] with one of the highest sea ice production rates [18] , and the consequent brine rejection promoted the formation of DSW [19] . Numerical modelling indicates that the DSW produced to the west of the MGT had the highest density and production rate for the 1992–2007 period among a number of coastal polynyas observed around East Antarctica [20] . However, dramatic changes to the region in January–February 2010, in particular, the calving of the MGT resulting from the positioning of iceberg B9b (ref. 21 ), have significantly altered the physical structure of the polynya system and raise important questions about the future of DSW formation and AABW production from this region. 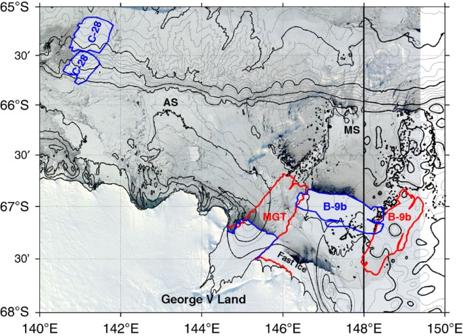Figure 1: Iceberg configuration. The MODIS/TERRA image from 22 April 201041showing icebergs C28 and B9b (labelled blue), with bathymetry and features. The previous configuration of MGT and B9b is shown in red. Figure 1: Iceberg configuration. The MODIS/TERRA image from 22 April 2010 [41] showing icebergs C28 and B9b (labelled blue), with bathymetry and features. The previous configuration of MGT and B9b is shown in red. Full size image Before the calving event, the MGT extended north across the Adélie Depression and was grounded on the continental shelf break southeast of the Mertz Bank ( Figs 1 and 2a ). Iceberg B9b was similarly positioned, but on the shallow bathymetry bounding the Mertz Depression to the east. After the calving event, Iceberg C28, the calved portion of the MGT, went away from the region, whereas B9b is stationary since the collision ( Figs 1 and 2a ). 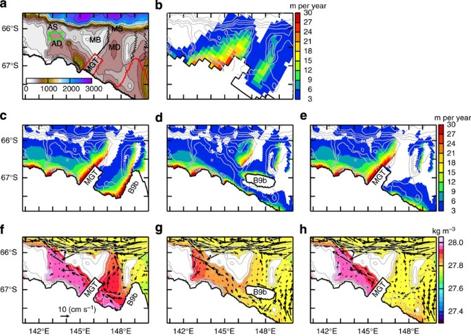Figure 2: Sea ice production and ocean circulation in the Adélie and the Mertz Depression regions. (a) Model bathymetry (colours and contours) for the region of interest and names for topographical features (AD, Adélie Depression; AS, Adélie Sill; MB, Mertz Bank; MD, Mertz Depression; MGT, Mertz Glacier Tongue; MS, Mertz Sill). Black points indicate the location of grounded icebergs in the model which block sea ice motion. (b) Satellite-based estimate for annual sea ice production (colours: annual rate of sea ice thickness growth per unit area). (c–e) Simulated annual sea ice production for CTRL, NOMGT and NOB9b. (f–h) Simulated current velocity (vectors) and seawater potential density (colours) at 425 m depth in September for CTRL, NOMGT and NOB9b. Bathymetry contours are also shown in (b–h). Figure 2: Sea ice production and ocean circulation in the Adélie and the Mertz Depression regions. ( a ) Model bathymetry (colours and contours) for the region of interest and names for topographical features (AD, Adélie Depression; AS, Adélie Sill; MB, Mertz Bank; MD, Mertz Depression; MGT, Mertz Glacier Tongue; MS, Mertz Sill). Black points indicate the location of grounded icebergs in the model which block sea ice motion. ( b ) Satellite-based estimate for annual sea ice production (colours: annual rate of sea ice thickness growth per unit area). ( c – e ) Simulated annual sea ice production for CTRL, NOMGT and NOB9b. ( f – h ) Simulated current velocity (vectors) and seawater potential density (colours) at 425 m depth in September for CTRL, NOMGT and NOB9b. Bathymetry contours are also shown in ( b – h ). Full size image Here, we assess the impact of the MGT calving event on dense water formation using a state-of-the-art ice-ocean model. From a series of numerical experiments, we found that the oceanic circulation and sea ice production in the Adélie and George V Land region changes immediately, and that the DSW export from the region is pronouncedly reduced. Outline of numerical experiments To assess the impacts of the MGT calving on DSW formation, numerical simulations of the Antarctic ice-ocean system are conducted under three configurations corresponding to the condition before the MGT calving event (case CTRL), the current scenario in which B9b resides at the current position (case NOMGT) and a likely future scenario about half a century later wherein B9b has also gone away but the MGT has extended again (case NOB9b) (see Methods for the detail of simulations). A case without either the MGT or B9b is also conducted but its result is not shown in this paper because it is essentially the same as NOMGT. Before the calving event The annual sea ice production over the Adélie and George V Land region is 339 km 3 in CTRL, 205 km 3 of which is produced to the west of the MGT and the rest (134 km 3 ) is produced to the east (the two regions are hereafter referred to as the Adélie Depression region and the Mertz Depression region, respectively). The sea ice production and ocean circulation in these regions are shown in Figure 2 . These numbers agree well with a satellite-based estimate [18] , which gives 194 km 3 for the Adélie Depression region and 116 km 3 for the Mertz Depression region. Sea ice production is especially high in the lee polynyas formed just to the west of the MGT and B9b ( Fig. 2b,c ). As the result of this intense sea ice production, waters as dense as 1,028 kg m −3 are produced under both polynyas in winter ( Fig. 2f ). The DSW formation in each region drives a flow along the northeastern (northwestern) edge of the Adélie (Mertz) Depression and a consequent outflow through the Adélie (Mertz) Sill. Shelf water dense enough to produce AABW flows out from each sill to the deep ocean ( Fig. 2f ). The volume fluxes of DSW (>1,027.80 kg m −3 ) outflow from the Adélie and the Mertz Sills are 0.35 and 0.31×10 6 m 3 s −1 , respectively ( Fig. 3 ). The corresponding rates of AABW production, prescribing the entrainment of ambient modified Circumpolar Deep Water (mCDW) during downslope mixing [20] , are 1.12 and 0.85×10 6 m 3 s −1 , respectively (see Methods for the estimation of AABW production). The modelled DSW outflow from the Adélie Depression and the corresponding AABW production are within the range of recent observational estimates [22] . 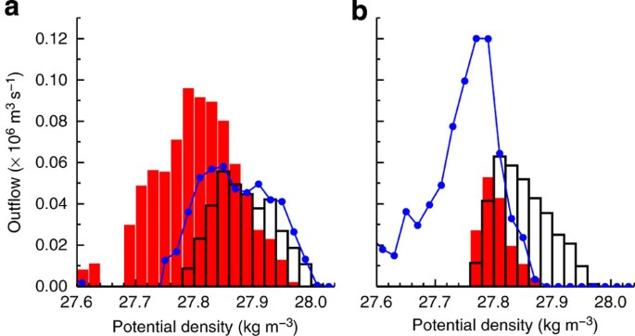Figure 3: Outflow of dense shelf water from the Adélie and the Mertz Depression regions. Volume flux (×106m3s−1) of outflowing water by 0.02 kg m−3incremented density classes. (a) Data are from the Adélie Depression and (b) from the Mertz Depression. CTRL case in black, NOMGT in red and NOB9b in blue. Figure 3: Outflow of dense shelf water from the Adélie and the Mertz Depression regions. Volume flux (×10 6 m 3 s −1 ) of outflowing water by 0.02 kg m −3 incremented density classes. ( a ) Data are from the Adélie Depression and ( b ) from the Mertz Depression. CTRL case in black, NOMGT in red and NOB9b in blue. Full size image After the calving event The removal of the MGT and repositioning of B9b markedly alter the sea ice production and oceanic circulation in the Adélie and the Mertz Depression regions. In NOMGT the annual sea ice production is reduced to 155 and 72 km 3 for the Adélie and the Mertz Depression regions, respectively, due mostly to the disappearance of the lee polynyas to the west of the MGT and B9b ( Fig. 2d ). Waters as dense as 1,028 kg m −3 are no longer found in these regions. A warm, less dense water flows into the Mertz Depression region from the east, which is absent in CTRL because of the blocking by B9b ( Fig. 2g ). Part of this water circulates within the Mertz Depression region and flows out through the Mertz Sill, and the rest flows into the Adélie Depression region and finally out through the Adélie Sill. As the density of this shelf water increases by the cumulative influence of brine rejection in the coastal polynyas along the George V coast and to the west of the grounded icebergs ( Fig. 2d ), the exported shelf water from the Adélie Depression is still sufficiently dense to form AABW ( Fig. 2g ). The outflowing volume flux of water denser than 1,027.80 kg m −3 from the Mertz Sill is drastically reduced to 0.08×10 6 m 3 s −1 . Conversely, the volume flux of the same density class from the Adélie Sill is increased to 0.43×10 6 m 3 s −1 because there is an inflow of water from the Mertz Depression region. The total outflow of DSW is reduced by 23% relative to CTRL. The mean density of outflow is also reduced for both sills: from 1,027.89 to 1,027.81 kg m −3 for the Adélie Sill and from 1,027.85 to 1,027.80 kg m −3 for the Mertz Sill. This magnitude of reduction is far from negligible, as the observed reduction in density over the continental slope around the Adélie and George V Land region is 0.009 kg m −3 per decade over the last 50 years [23] , whereas the modelled change due to the calving of MGT, 0.05 kg m −3 , occurs abruptly in the first winter. The rates of AABW production for NOMGT are 1.41 and 0.20×10 6 m 3 s −1 for the Adélie and the Mertz Depression regions, respectively. The total reduction relative to CTRL, 0.36×10 6 m 3 s −1 (18 %), is also non-negligible. Future scenario In a potential long-term future scenario wherein B9b eventually migrates away from the region and the floating extension of the MGT reforms, DSW outflow from the Adélie and the Mertz Depression regions is partly restored. Sea ice production, DSW formation and oceanic circulation in the Adélie Depression region for NOB9b ( Fig. 2e,h ) are basically the same as those for CTRL, and the outflow of DSW is almost restored to the situation of CTRL ( Fig. 3a ). However, the water in the Mertz Depression region is further reduced in density because the absence of B9b reduces sea ice production and the re-emergence of the MGT decreases the transport of less dense water from the east into the Adélie Depression, re-establishing the circulation within the Mertz Depression region and flow out from the Mertz Sill ( Fig. 2e,h ). The volumetric outflow from the Mertz Sill increases considerably, but the DSW portion is almost the same as in NOMGT ( Fig. 3b ). The total outflowing volume flux of water denser than 1,027.80 kg m −3 from the Adélie and Mertz Sills is 0.55×10 6 m 3 s −1 and the corresponding AABW production is estimated to be 1.75×10 6 m 3 s −1 , about an 11% reduction relative to CTRL. The DSW formation and export in CTRL exhibit a long-term trend and interannual variability. The potential density just south of the Adélie Sill decreases at a rate of 0.013 kg m −3 per decade, and the s.d. of its interannual variation is 0.021 kg m −3 ( Fig. 4a ). The MGT calving event has pronounced impact on the DSW properties when compared with the natural variability. The event also influences export of DSW from the Adélie and the Mertz Depressions ( Fig. 4b,c ). Note that the long-term trend in CTRL is not due to model climate drift but a response to variability in the atmospheric forcing, as the model climate does not have a notable trend during the spin-up stage. 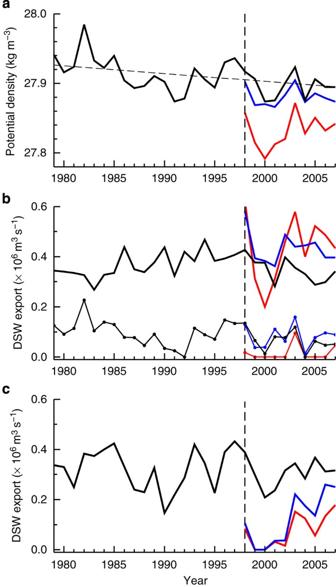Figure 4: Time series of dense shelf water (DSW) properties. (a) Annual mean potential density (kg m−3) just south of Adélie Sill (see green box inFig. 2afor the location). (b) Dense shelf water export (×106m3s−1) from the Adélie Depression. (c) Dense shelf water export from the Mertz Depression. In (b,c) thick lines show the export of water denser than 1,027.80 kg m−3. In (b) thin lines with dots show the export of water denser than 1,027.94 kg m−3. CTRL case in black, NOMGT in red and NOB9b in blue. Vertical dashed line indicates start time for NOMGT and NOB9b cases. Figure 4: Time series of dense shelf water (DSW) properties. ( a ) Annual mean potential density (kg m −3 ) just south of Adélie Sill (see green box in Fig. 2a for the location). ( b ) Dense shelf water export (×10 6 m 3 s −1 ) from the Adélie Depression. ( c ) Dense shelf water export from the Mertz Depression. In ( b , c ) thick lines show the export of water denser than 1,027.80 kg m −3 . In ( b ) thin lines with dots show the export of water denser than 1,027.94 kg m −3 . CTRL case in black, NOMGT in red and NOB9b in blue. Vertical dashed line indicates start time for NOMGT and NOB9b cases. Full size image The total AABW production rate around Antarctica remains poorly quantified and controversial, with the estimates ranging between 10 and 15×10 6 m 3 s −1 (refs [24] –26). It is currently suggested that 60% of the total AABW is formed in the Weddell Sea and the rest is formed in the Ross Sea and Adélie and George V Land region [4] . The AABW from the Adélie and George V Land region, in conjunction with AABW from the Ross Sea, ultimately supplies to the abyssal layers of the eastern Indian and Pacific oceans [4] , [14] , [27] , influences the variability of their abyssal layers. We estimate that the 0.36×10 6 m 3 s −1 reduction in AABW from the Adélie and George V Land region found in this study leads to about 6–9% reduction in the AABW of these ocean basins. However, the present model is not optimal for quantifying the impact of the MGT calving on the abyssal World Ocean and global thermohaline circulation, in particular with respect to downslope mixing of DSW overflow on the continental shelf and lacks the global resolution to assess all DSW formation sites outside of the Adélie and George V Land region. Here, we try to speculate on its potential impact. A recent data-assimilating modelling [15] indicates that the origin of the observed warming in the abyssal North Pacific Ocean over the recent decade [7] can be traced back to a change of dense water formation off the Adélie and George V Land coast. Although the renewal timescale of the abyssal ocean water masses is millennial or longer, the initial dynamical response of the thermohaline circulation to changes in deep water formation appears over a decadal timescale as its effect propagates by relatively fast Kelvin and Rossby waves [28] , [29] . As the magnitude of the change in dense water formation off the Adélie and George V Land coast by the MGT calving is comparable to its past decadal changes ( Fig. 4a ), the MGT calving could induce a change in the abyssal North Pacific Ocean whose magnitude is comparable to the observed recent decadal change. Further quantification of these potential changes necessitates an increased sophistication in future models. There is observational evidence that the dense water formed in the Ross Sea comparably contributes to the bottom layer water in the North Pacific Ocean [4] . Although the above-mentioned data-assimilating modelling does not point to the importance of the Ross Sea, ocean models, especially of coarse resolution, are not yet free from problems in simulating total deep water formation around Antarctica and its migration into the North Pacific Ocean [30] . The dynamic nature of the Antarctic ice front, through the periodic calving of continental ice shelves/glaciers, and the subsequent migration/grounding of the icebergs formed is likely to be a major component of the multi-decadal variability of polynya regions and the DSW formation therein for AABW production. The current modelling results suggest that the DSW is modulated by such changes. The local change of dense water induced by the present MGT calving event is expected to be at least comparable to observed changes resulting from climate changes over the previous couple of decades [31] , [32] , [33] . Decadal to multi-decadal changes in dense water formation and associated global ocean circulation may also be controlled by such events. In this regard, we must investigate further the behaviour of glacier tongues/ice shelves and the oceanic response to better our understanding and prediction of the long-term variability of the global ocean and climate. Ice-ocean model The numerical ice-ocean model used here is based on COCO [34] . The oceanic part of the model is a z -coordinate general circulation model, and the sea ice part uses one layer thermodynamics [35] , a two category thickness representation [36] , and an elastic-viscous-plastic rheology [37] . The model domain is global, and its horizontal curvilinear grid is set up so that the horizontal grid size is <5 km over the Adélie and George V Land region and <15 km over the entire East Antarctic continental shelf [20] . There are 69 vertical levels: 5 of which are in the top 50 m; the vertical spacing between 50 m depth and 1,500 m depth is 50 m; and that below 1,500 m depth is 100 m. The blocking of sea ice motion by grounded icebergs is accounted for [20] (see Fig. 2a for their locations). This model has been shown to effectively reproduce the coastal polynyas, ice production [20] , ocean circulation around the Adélie and George V Land region, a dual-system for DSW formation and export from Adélie and the Mertz Depressions (Kusahara et al ., unpublished manuscript), which is consistent with recent observational analysis over the continental slope and rise [13] . Experiments The ice-ocean model is first integrated for 18 years by prescribing daily climatological atmospheric conditions [38] to obtain a quasi-steady state. Initiated by this state, a simulation is carried out for the period of 1979–2007 using daily reanalysis atmospheric conditions [39] under the pre-MGT-calving condition (case CTRL; Fig. 2c ). Two 10-year calculations are conducted from January 1998 of CTRL. In the current/short-term future the calved MGT has migrated away from the region, whereas B9b remains in its new position. Case NOMGT deals with such a near-future situation ( Fig. 2d ). In the longer-term B9b is also expected to break apart and leave the region. On the other hand, the MGT is extending at a rate of ∼ 1 km per year (ref. 21 ) and will re-extend to the pre-calving configuration in about half a century. Case NOB9b deals with such a later situation ( Fig. 2e ). The lines of small-grounded icebergs extending from the tip of the MGT and B9b of the pre-calving situation remain in NOMGT and NOB9b. Data from the last 10 years of the simulations are used for the present analyses unless otherwise noted. The results of sea ice production, DSW export (defined by specific cutoff potential densities 1,027.80, 1,027.88 and 1,027.94 kg m −3 ) and estimated AABW production in the three experiments are summarized in Table 1 . Table 1 Summary of sea ice production, dense shelf water export and estimated AABW production in the three experiments. Full size table Estimation of AABW production Using the potential temperature-salinity characteristics of the outflowing DSW, we estimate the AABW production under the following three assumptions [20] . First, the AABW is a mixture of the outflowing DSW and mCDW over the continental slope. Second, the properties of mCDW lie between 1,028.00 and 1,028.27 kg m −3 in neutral density ( γ n , ref. 40 ) and between 0.2 and 1.0 °C in potential temperature (grey shaded area in Fig. 5 ). Third, all outflowing waters denser than γ n =1,028.27 kg m −3 and lower than 0.0 °C mix with the prescribed mCDW and form uniform AABW of γ n =1,028.27 kg m −3 . In other words, the water mass properties of the estimated AABW are determined by the intersection between the neutral density curve or the zero potential temperature line (green curve in Fig. 5 ) and mixing line that connects the two water mass characteristics in potential temperature-salinity space. The mixing ratio of the outflowing DSW to the prescribed MCDW is given by the ratio of distances between the intersection of AABW (green line in Fig. 5 ) and the mixing line between source waters in temperature-salinity space. 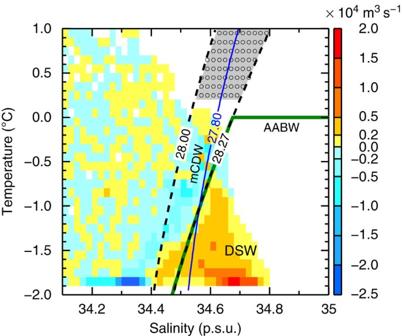Figure 5: Outflow and inflow in the potential temperature-salinity space. Outflow and inflow are estimated by the volume flux across the northern boundary of the Adélie Depression. Bin intervals for potential temperature (vertical axis) and salinity (horizontal axis) are 0.1 °C and 0.02 p.s.u., respectively. Positive (negative) values (represented in the colour bar) show outflow from (inflow into) the Adélie Depression. Dashed black and solid blue lines are neutral density surfaces (γn=1,028.00 and 1,028.27 kg m−3) and the potential density (σθ=1,027.80 kg m−3), respectively. The green line shows the boundary of the AABW. Grey area shows the property of the prescribed mCDW, and circles therein indicate sampled points for the estimation of AABW production. Figure 5: Outflow and inflow in the potential temperature-salinity space. Outflow and inflow are estimated by the volume flux across the northern boundary of the Adélie Depression. Bin intervals for potential temperature (vertical axis) and salinity (horizontal axis) are 0.1 °C and 0.02 p.s.u., respectively. Positive (negative) values (represented in the colour bar) show outflow from (inflow into) the Adélie Depression. Dashed black and solid blue lines are neutral density surfaces ( γ n =1,028.00 and 1,028.27 kg m −3 ) and the potential density ( σ θ =1,027.80 kg m −3 ), respectively. The green line shows the boundary of the AABW. Grey area shows the property of the prescribed mCDW, and circles therein indicate sampled points for the estimation of AABW production. Full size image How to cite this article: Kusahara, K. et al . Impact of the Mertz Glacier Tongue calving on dense water formation and export. Nat. Commun. 2:159 doi: 10.1038/ncomms1156 (2011).